Persistent drying in the tropics linked to natural forcing Approximately half of the world's population lives in the tropics, and future changes in the hydrological cycle will impact not just the freshwater supplies but also energy production in areas dependent upon hydroelectric power. It is vital that we understand the mechanisms/processes that affect tropical precipitation and the eventual surface hydrological response to better assess projected future regional precipitation trends and variability. Paleo-climate proxies are well suited for this purpose as they provide long time series that pre-date and complement the present, often short instrumental observations. Here we present paleo-precipitation data from a speleothem located in Mesoamerica that reveal large multi-decadal declines in regional precipitation, whose onset coincides with clusters of large volcanic eruptions during the nineteenth and twentieth centuries. This reconstruction provides new independent evidence of long-lasting volcanic effects on climate and elucidates key aspects of the causal chain of physical processes determining the tropical climate response to global radiative forcing. An overall intensification of the global hydrological cycle is generally reported to occur under a warming climate [1] . How such general intensification affects regional rainfall regimes and eventually the distribution of available freshwater, however, strongly depends on associated large-scale atmospheric circulation changes [1] . Mesoamerica, the stretch of land separating the tropical Atlantic and tropical Pacific oceans ( Fig. 1a ), is considered to be the tropical region most exposed to climate change and subject to substantial drying in the future according to climate projections [2] . To increase our confidence in projected drying scenarios, it is incumbent to improve our understanding of the causes and forcing mechanisms of this region’s long-term hydroclimate variability, also based on information from the remote past. 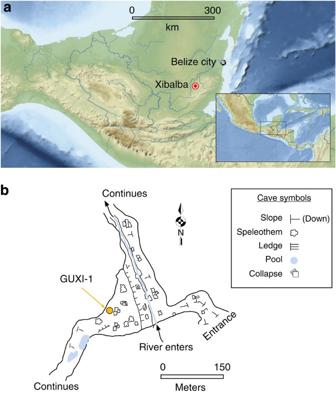Figure 1: Geographical characteristics of the study area. (a) Location map of Mesoamerica and of the Xibalba cave; (b) Map of the speleothem site with major physical features of the cave. Figure 1: Geographical characteristics of the study area. ( a ) Location map of Mesoamerica and of the Xibalba cave; ( b ) Map of the speleothem site with major physical features of the cave. Full size image The climate of Mesomerica ( Fig. 1a ) is characterized by a boreal summer/fall (June–October) rainy season and a relatively dry winter [3] . Mesoamerica’s rainfall is influenced by moisture originating usually from the vicinity of the Intertropical Convergence Zone (ITCZ) via transport into the monsoonal system over Belize, via the Caribbean low-level jet, and by localized convection. In summer, the ITCZ migrates to its northern position, its core stretching across the northern tropical Atlantic at ∼ 10°N, into northern South America and from there turning north over Central America to the East Pacific, reaching to ∼ 12°N and causing widespread rainfall over the land portion [4] . Because the two ITCZ segments respond to variations in sea-surface temperatures (SSTs) in both the tropical Atlantic and the Pacific Oceans, Mesoamerica is exposed to complex hydrological fluctuations on a broad range of timescales [5] . Year-to-year rainfall variability in the Guatemala mountain regions today is correlated with the gradient between SSTs in the western tropical Atlantic and eastern tropical Pacific [3] . Colder (warmer) than normal tropical Atlantic SSTs that are consistent with a stronger (weaker) and more southward (northward) displaced Atlantic subtropical high, lead to drier (wetter) than normal conditions in Central America [6] , [7] . Similarly, anomalously warm (cold) eastern equatorial Pacific SSTs, e.g., during El Niño (La Niña) events, force an equatorward (northward) displacement of the east Pacific ITCZ and contribute to drying (wetting) in most of Central America [8] , [9] . Observations also indicate an association between precipitation conditions over Mesoamerica and the phasing of the winter North Atlantic Oscillation [10] . Timing and distribution of precipitation during the summer season is a critical issue for agricultural yields in Yucatán: periods of drought vitally affect agriculture and, hence, local societies [11] . Observational meteorological records indicate that droughts on the peninsula are rare, but tend to be more severe than wet periods [11] . The availability of continuous, long-term hydrological data beyond the few decades covered by the instrumental record is a necessary prerequisite to fully characterize regional hydrological variability and to unequivocally address its dependence on large-scale climatic fluctuations, especially as far as the identification of forcing mechanisms at the hemispheric to global scales is concerned. Elucidation of Mesoamerican hydroclimate variability and associated dynamics before the instrumental period will also contribute to the debate on the intricate cultural changes that occurred in the region during pre-Columbian times [12] . Speleothems are increasingly used as terrestrial archives of past climate and environmental change because they can provide long, continuous, precisely U-series dated and high-resolution time series, and are generally unaffected by post-depositional diagenetic alteration. Here we present results from a new 300 year (1700–2000 C.E.) precipitation reconstruction based on δ 18 O from a Mesoamerican speleothem. Our paleo-precipitation data reveal large multi-decadal declines in regional precipitation, the onset of which coincide with clusters of large volcanic eruptions. Our data show, for the first time, that natural external forcing can drive successive multi-decadal dry and wet phases in the tropics and provide new independent evidence of long-lasting tropical climate response to global radiative forcing, contributing to the current debate on whether strong tropical volcanic eruptions and changing solar output have the potential to induce dynamical responses in the coupled ocean–atmosphere system on decadal and even longer time scales. Hydrological reconstruction and volcanic eruptions The data for this study derive from stalagmite GU-Xi-1 collected 250 m inside the large cavern of Xibalba in the Campur Formation [13] located in the Maya Mountains of Guatemala near the Belize border ( Fig 1a , 16.5°N, 89°W). The in-cave elevation is 350 m, with a cave mean annual temperature of 23 °C. GU-Xi-1 was actively dripping at the time of collection and chosen for its candle-shape, its distance from outside atmospheric influences, and its location of 30 m above the nearby modern river level; the karst surface is generally 100–150 m above the cave passages ( Fig. 1b ). The specimen is 33 cm tall, but only the upper 18 cm are used for this study ( Fig. 2a ). Our age model ( Fig. 2b ) is highly constrained by nine U/Th multi-collector inductively coupled plasma mass spectrometry dates ( Supplementary Table 1 ) and by the collection date in 2007. 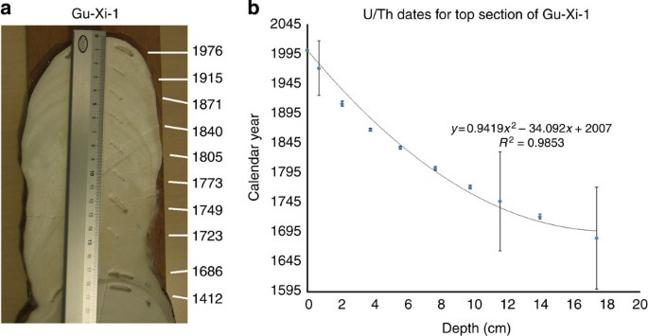Figure 2: Image of the speleothem and age model. (a) The photograph of GU-Xi-1 stalagmite shows the height of the specimen used in this study (18 cm), with a rounded top and no ‘cup’ that could imply drip erosion. Also shown is the milling channel for the stable isotopes adjacent to a cm ruler as well as the upper nine pits on stalagmite GU-Xi-1 (upper part) used to for age determination. (b) Age model that we used in this study. A thorough discussion on the age model is presented in the methods section. The vertical lines represent the error bars (two s.d.). Figure 2: Image of the speleothem and age model. ( a ) The photograph of GU-Xi-1 stalagmite shows the height of the specimen used in this study (18 cm), with a rounded top and no ‘cup’ that could imply drip erosion. Also shown is the milling channel for the stable isotopes adjacent to a cm ruler as well as the upper nine pits on stalagmite GU-Xi-1 (upper part) used to for age determination. ( b ) Age model that we used in this study. A thorough discussion on the age model is presented in the methods section. The vertical lines represent the error bars (two s.d.). Full size image The largest amounts of annual precipitation in the region fall on the high mountain ranges of Guatemala, southwest of the cave. Summer precipitation values in the Maya Mountains reach upwards of 400 mm per month, but are approximately half that amount in the study area. A strong inverse correlation between speleothem δ 18 O and tropical precipitation intensity [14] has previously been observed for the region [15] . The speleothem δ 18 O significantly correlates (see methods) with precipitation from nearby Belize City over the instrumental period, when a lag of 6 years is imposed to the former ( Fig. 3 ). The inverted correlation patterns of the speleothem δ 18 O with the SST and sea-level pressure (SLP) fields over the Pacific and Atlantic sectors is consistent with corresponding patterns for observed precipitation ( Fig. 4 ), supporting the robustness of the climatological scenario associated with interannual rainfall variability over the Yucatán. 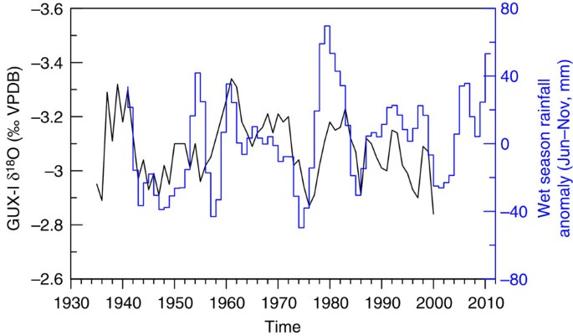Figure 3: Comparison between reconstructed and observed Mesoamerican precipitation. Shown are the time series of speleothem GU-Xi-1 δ18O (black line, units in permil) and June–November precipitation anomalies in Belize City, Belize (deviation from climatology in mm, blue line) smoothed with a second order binomial filter. The δ18O time series lags the rainfall time series by 6 years. Figure 3: Comparison between reconstructed and observed Mesoamerican precipitation. Shown are the time series of speleothem GU-Xi-1 δ 18 O (black line, units in permil) and June–November precipitation anomalies in Belize City, Belize (deviation from climatology in mm, blue line) smoothed with a second order binomial filter. The δ 18 O time series lags the rainfall time series by 6 years. 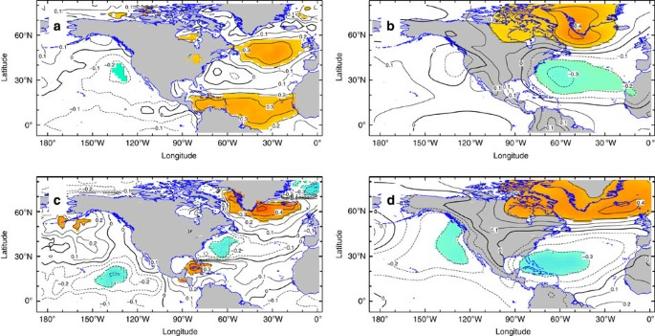Figure 4: Atmosphere and ocean relationships to Mesoamerican rainfall. (a,b) Correlations between summertime (May–October) observed precipitation averaged over the Yucatán Peninsula and SST (a) and SLP (b). (c,d) Correlations of the SST and SLP fields with the GU-Xi-1 speleothem δ18O (multiplied by −1). Contours in all figures are drawn at 0.1 intervals. Regions where the correlation exceeds the 95% confidence level for significance are shaded in colour (orange for positive and light blue for negative). Full size image Figure 4: Atmosphere and ocean relationships to Mesoamerican rainfall. ( a , b ) Correlations between summertime (May–October) observed precipitation averaged over the Yucatán Peninsula and SST ( a ) and SLP ( b ). ( c , d ) Correlations of the SST and SLP fields with the GU-Xi-1 speleothem δ 18 O (multiplied by −1). Contours in all figures are drawn at 0.1 intervals. Regions where the correlation exceeds the 95% confidence level for significance are shaded in colour (orange for positive and light blue for negative). Full size image The most prominent aspects of our reconstruction are the occurrences of three distinct multi-decadal drying trends during the nineteenth and twentieth centuries ( Fig. 5e ). Based on the modern relationship between δ 18 O and regional precipitation anomalies [16] , the speleothem data indicate a 25% decrease in precipitation between 1810 and 1845 C. E., another comparable precipitation decrease between 1883 and 1925 C. E., and a third, smaller decrease from 1963 to the present. The drying steps are separated from one another by brief intervals of precipitation recovery in mid-century. Our and other available δ 18 O records from Mesoamerica [17] , [18] correlate with each other with variable strength during the reconstruction period ( Fig. 6 , Supplementary Figs 1, 2 ), in part reflecting large dating uncertainties in some of the reconstructions. The different reconstructions feature similar drying trends during the early and—less so—late nineteenth century, suggesting a broader regional phenomenon. 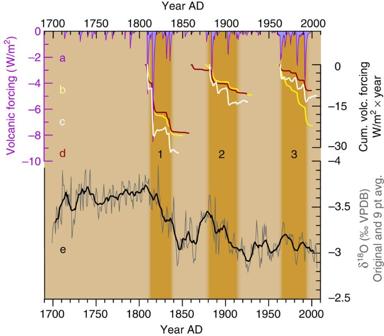Figure 5: Persistent drying phases over Mesoamerica and volcanic forcing. (a) Volcanic radiative forcing from 1700–2000 C. E. after ref.28. Dark vertical shaded areas indicate volcanic eruption clusters noted in the text. (b–d) Different estimates of cumulative top-of-atmosphere radiative flux anomalies from different climate simulations: Bergen Climate Model (Fig. 5b, yellow), CCSM4 (Fig. 5c, white) and ECHAM5/MPIOM (Fig. 5d, brown). (e) Interpolated annual time series of speleothem GU-Xi-1 δ18O (grey line) with corresponding 11-year moving average values (thick black line). Figure 5: Persistent drying phases over Mesoamerica and volcanic forcing. ( a ) Volcanic radiative forcing from 1700–2000 C. E. after ref. 28 . Dark vertical shaded areas indicate volcanic eruption clusters noted in the text. ( b – d ) Different estimates of cumulative top-of-atmosphere radiative flux anomalies from different climate simulations: Bergen Climate Model ( Fig. 5b , yellow), CCSM4 ( Fig. 5c , white) and ECHAM5/MPIOM ( Fig. 5d , brown). ( e ) Interpolated annual time series of speleothem GU-Xi-1 δ 18 O (grey line) with corresponding 11-year moving average values (thick black line). 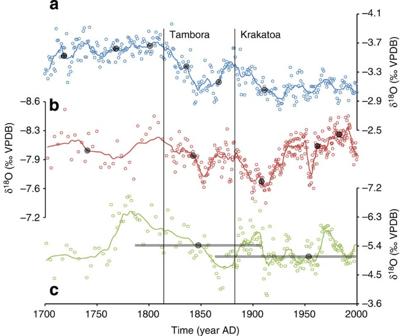Figure 6: Comparison between stalagmite records from Mesoamerica. (a) GU-Xi-1 (this study); (b) southwestern Guerrero (Mexico)17; and (c) Yucatán peninsula (Mexico)18. Open circles represent the raw data from each record. Solid lines represent the 5-point running average applied to the series. The grey circles represent the locations from which the material for the U/Th dates were obtained and the control points of the age models used. The horizontal grey bars represent the uncertainty of each age control point. The difference in alignments of these records depends on their age models (note poor age control of the Yucatán record18) sampling resolution and extent of local and cave environmental overprinting. Full size image Figure 6: Comparison between stalagmite records from Mesoamerica. ( a ) GU-Xi-1 (this study); ( b ) southwestern Guerrero (Mexico) [17] ; and ( c ) Yucatán peninsula (Mexico) [18] . Open circles represent the raw data from each record. Solid lines represent the 5-point running average applied to the series. The grey circles represent the locations from which the material for the U/Th dates were obtained and the control points of the age models used. The horizontal grey bars represent the uncertainty of each age control point. The difference in alignments of these records depends on their age models (note poor age control of the Yucatán record [18] ) sampling resolution and extent of local and cave environmental overprinting. Full size image Our three pronounced decreases in regional precipitation coincided with clusters of strong tropical volcanic eruptions ( Fig. 5a ). The most prominent of these eruptions are the 1809 eruption of unknown location and Tambora in 1815 (cluster 1), Krakatau in 1883 (cluster 2), Agung in 1963 and Pinatubo in 1991 (cluster 3). Reconstructed precipitation decreases throughout each cluster such that the precipitation evolution during these periods is best described as a function of cumulative volcanic radiative forcing ( Figs 5b–d , Supplementary Figs 3, 4 and Supplementary Note 1 ). The different estimates of cumulative volcanic forcing provided in Fig. 5 exemplify the effects of uncertainties, such as those in reconstructed aerosol optical properties used as volcanic forcing input to climate models, those arising from the presence of additional varying external forcing factors and those inherent in the model-specific implementation of volcanic forcing. The most recent volcanic cluster does not display a statistically significant correlation between δ 18 O and cumulative volcanic forcing, that we interpret as the result of the different background climate conditions and of interferences from other dominant forcing factors during the mid- to late-twentieth century. For the nineteenth century clusters, the drying trend only reverses when volcanic activity substantially weakens. The precipitation recovery is only partial, possibly as part of recurrent drying trends in Mesoamerica [15] , [19] . Aerosols are a known critical part of the overall anthropogenic as well as natural forcing of climate (the latter associated with aeolian dust and volcanic eruptions) [20] , [21] , [22] . We thus surmise that the decadal drying trends in the early and late decades of the nineteenth century and during the second half of the twentieth century are largely a consequence of the clustered volcanic forcing, with the most recent period superposed on long-term anthropogenic drying [23] , [24] . Periods of strong volcanic activity during the past millennium also often coincide with periods of anomalous solar activity. This is the case, for instance, for the first volcanic cluster that coincides with the prolonged period of weak solar activity known as Dalton Minimum [25] . We can thus not attribute the reconstructed changes to volcanic forcing alone. Dynamical interpretation of reconstructed changes Based on the close agreement between the drying phases and the volcanic clusters, we hypothesize that the eruption clusters played a primary role in these climatic changes by inducing perturbations in patterns of SST variability that in turn crucially influence the Pacific–Atlantic tropical SST gradient that dominate the Mesoamerican hydroclimate. Specifically, we propose that the volcanic clusters influence the El Niño Southern Oscillation (ENSO) in the equatorial Pacific and the long-term variations of tropical Atlantic SSTs, which is governed by the Atlantic Multi-decadal Oscillation (AMO) [26] . An increasing number of climate reconstructions and simulations describe statistical and dynamical connections between volcanic forcing and both ENSO [27] and AMO [28] , [29] , [30] . Indeed, drying (recovery) phases during the volcanic clusters correspond to cold (warm) phases in a recent marine proxy-based AMO reconstruction [31] ( Fig. 7a ), while reconstructed data [32] suggest an increased role for ENSO in Mesoamerican precipitation variability during the twentieth century ( Fig. 7b ). The preferred time scales of significant coherence with the δ 18 O signal differ between ENSO and AMO, as the former index highlights interdecadal time scales (O(30 years)), while the latter highlights multi-decadal time scales (O(50 years)), further suggesting that the linkages may reflect different teleconnection mechanisms (see also Fig. 7c ). Such differences in the relative roles of climatic modes indicate that internal dynamics play a substantial role in communicating high atmospheric evolution during the different volcanic eruption clusters to the surface. This exemplifies the complexity of a dynamical interpretation, and hence attribution, of the reconstructed changes in Mesoamerican precipitation. Moreover, reconstructions of climate modes often lack robustness due to the inherent uncertainties implicated in reconstructing large-scale features from a limited number of local climate proxies. This has been shown for the North Atlantic Oscillation [33] that captures a dominant part of the short- and long-term variability of large-scale atmospheric circulation over the North Atlantic, which is a known factor influencing Mesoamerican precipitation ( Figs 4b,d ) and is sensitive to volcanic forcing [34] , [35] . 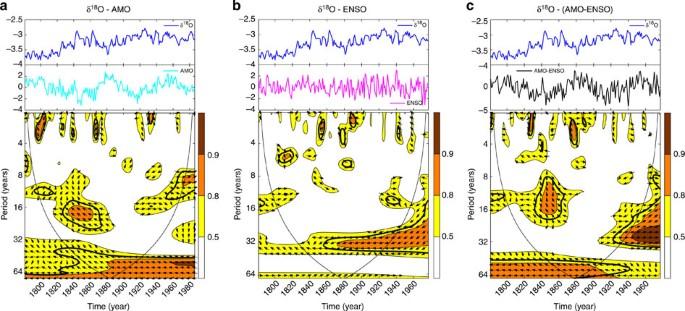Figure 7: Linkage between reconstructed Mesoamerican precipitation and dominant modes of climate variability. The different panels show wavelet coherences (power in colour shading) between the speleothem δ18O and: (a) the AMO reconstruction by Svendsenet al.31; (b) the integrated ENSO/PDO reconstruction by ref.32; and (c) the difference between the two. The time series are shown in the top and middle panels (blue: δ18O; turquoise: AMO; magenta: ENSO; black: difference between AMO and ENSO). The arrows illustrate the phase relationship: rightward (leftward) arrows indicate co-phase (anti-phase); northward and southward oriented arrows indicate quadrature. Thick contour lines identify significant62coherence. The thin black lines are the cone of influence, where edge effects occur. Figure 7: Linkage between reconstructed Mesoamerican precipitation and dominant modes of climate variability. The different panels show wavelet coherences (power in colour shading) between the speleothem δ 18 O and: ( a ) the AMO reconstruction by Svendsen et al. [31] ; ( b ) the integrated ENSO/PDO reconstruction by ref. 32 ; and ( c ) the difference between the two. The time series are shown in the top and middle panels (blue: δ 18 O; turquoise: AMO; magenta: ENSO; black: difference between AMO and ENSO). The arrows illustrate the phase relationship: rightward (leftward) arrows indicate co-phase (anti-phase); northward and southward oriented arrows indicate quadrature. Thick contour lines identify significant [62] coherence. The thin black lines are the cone of influence, where edge effects occur. Full size image A warranted dynamical interpretation based on modelling results is also complicated by the fact that last-millennium simulations from state-of-the-art global climate models do not show a consistent response of Mesoamerican precipitation to strong volcanic activity ( Fig. 8 ), failing to robustly reproduce the patterns reconstructed from our speleothem. The discrepancy between our reconstruction and the simulations can be ascribed to general deficiencies still affecting the simulated representation of key chemical and physical processes related to aerosol forcing, and to the consequent large uncertainties in the simulated climate response to volcanic forcing [25] , [36] . Further possible explanations are the common model deficiencies concerning regional precipitation variability at the decadal and multi-decadal time scales [37] , which are linked to poor and hence less robustly simulated representation of dominant modes of large-scale climate variability and associated teleconnections including ENSO [38] and the AMO [39] . Large uncertainties also affect the reconstructed forcing [40] and we have very limited knowledge about the background climate conditions at the time of volcanic eruptions that occurred before the last half of the twentieth century [30] . 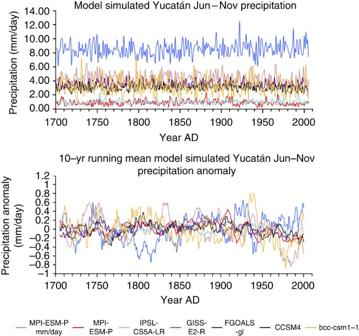Figure 8: June–November precipitation in Yucatán from Coupled Model Intercomparison Project 5 simulations covering the period 1700–2005. (a) Raw time series, (b) 10-year running mean, where the climatological mean has been subtracted. Figure 8: June–November precipitation in Yucatán from Coupled Model Intercomparison Project 5 simulations covering the period 1700–2005. ( a ) Raw time series, ( b ) 10-year running mean, where the climatological mean has been subtracted. Full size image The prolonged post-eruption drying conditions in Mesoamerica described by our new speleothem-based data provide independent evidence that volcanic effects on tropical climate persist well beyond the duration of the direct radiative imbalance [35] . We suggest that volcanically induced changes in dominant modes of large-scale, ocean–atmosphere coupled variability is a likely physical mechanism contributing to such persistence. Further studies are needed to clarify the dynamics governing the response. Still, our observation relating clusters of large volcanic eruptions to prolonged decreased Mesoamerican precipitation should expand the emerging discussion fostered by indications from global climate models regarding the strong sensitivity of the world’s other monsoons to external forcing [41] , [42] . Our results, in combination with studies of global stream flows after large volcanic eruptions [43] , imply that certain tropical hydroclimates may be highly sensitive to volcanic forcing and, more generally, to large stratospheric aerosols loading [24] . Global climate models have become increasingly important to our physical understanding of such ‘global forcing to regional response’ connections. As discussed, however, related uncertainties affecting the simulated representation (or lack thereof) of key processes as well as the reconstructed external forcing that is imposed on paleo-simulations remain considerable. We need to better understand such critical aspects of reconstructed as well as simulated pre-industrial tropical climate evolution in order to increase our confidence in projected future regional precipitation trends and variability and to potentially customize solutions for particular regions. Speleothem characteristics and analysis We collected the GU-Xi-1 stalagmite in 2007 from the Xibalba cave located in a thick forest near the Guatemala/Belize border ( Fig. 1b ), and mapped its underground location relative to the surface. The ceiling height varies from 10 m to >40 m. The collection site lies well above the level of modern floods, which eliminates inaccuracies in dating due to possible initial detrital 230 Th. GU-Xi-1 was active and growing at the time of collection, with a columnar shape indicating it was a product of a single-drip source. The stalagmite was cut into two sections and a 1-cm thick slab was produced from one of the sections. Age model An amount of 200 mg of powder was collected with a hand-held dental drill from a polished slab section of GU-Xi-1 along growth layers for dating. Nine 230 Th dates were analyzed in the upper 175 mm resulting in an age control point approximately every 30 years ( Fig. 2a ). We analyzed three samples for thorium and uranium isotopes separately on a Finnigan-MAT Element outfitted with a double focusing sector field magnet in reversed Nier–Johnson geometry and a single Mas Com multiplier. We measured combined ionization plus transmission efficiency of 2.5–3% for uranium and 1.5–2% for thorium. Dating resolution using the machine was 40–80 years. Six more samples were analyzed with a Neptune ICP-MS MC, with a dating resolution of <4 years. Further details of instrumental procedures are explained in refs 44 , 45 . We obtained these dates with a magnetic sector inductively-coupled plasma mass spectrometer at the University of Minnesota, Isotope Laboratory [46] . Chemical separation procedures followed those described in ref. 47 . The age model for the speleothem is based on a parabolic curve fit to the 230 Th dates and the collection date ( Fig. 2b ). Error bars are larger for the ages determined with a Finnigan-MAT Element compared with the dating resolution obtained using the Neptune ICP-MS MC ( Fig. 2b ). We used AnalySeries ( http://www.lsce.ipsl.fr/logiciels/index.php ) to regress the U/Th ages with depth. We found that the upper section of GU-Xi-1 grew according to a second-degree polynomial that was parabolic ( r =0.99). We removed any sampling bias with AnalySeries using the integration method to provide evenly spaced annual samples. We used the resulting polynomial equation to convert each sample depth to calendar ages from the speleothem, which we used for our age model. Different possible age models have been tested ( Supplementary Fig. 5 ), including StalAge [48] , COPRA [49] , calcium (Ca) layer counting and the average between StalAge and the Ca count methods (ChronMean). All the tested models agree closely with the timing of the drying event observed from the stable isotope record associated with the Tambora eruption. The largest uncertainty is the timing of the Krakatau eruption. It should be noted that because GU-Xi-1 growth slowed down considerably towards the present (from 1915 to 2007 it grew 2.5 times slower than from 1840 to 1871) any error for the more recent samples in assigning a depth to a U/Th date is exacerbated. StalAge is a routinely used algorithm specifically designed for speleothems. It takes into account outliers and age inversions using a Monte Carlo simulation. In our case, as we do not have outliers or age inversions, it basically performs a linear interpolation between age points. A similar age model [49] gives near identical results to that of StalAge. Another approach is to count the annual laminations (clearly present in GU-Xi-1). We are confident the laminations are annual because the number of laminations counted is within 97% confidence limits of the U/Th dates. The annual layers are tedious to count and also produce subjective counting errors. Another more objective method is to count the number of annual Ca peaks that clearly follow the annual banding. During summer more Ca is incorporated in the speleothems [50] . The results from this method are shown as the Ca counts chronology in Supplementary Fig. 1 and clearly lie to the right (younger) side of the age model especially from 1830 to the present. According to StalAge the ‘Krakatau’ event (as seen in the stable isotopes) occurred in 1864 (about 20 years earlier) but according to the Ca counts the event occurred in 1910 (about 20 years later). StalAge based on U/Th dates may be biased towards recent samples because of the greater uncertainties (5–10% of the absolute age [51] ) for younger speleothems with low U, thus limiting the possibility to correlate time-series based on speleothems with those based on instruments. A further approach is to take the mean of both the StalAge and the Ca count methods. The mean is shown as the ‘ChronMean’ in Supplementary Fig. 5 . The ChronMean model also smoothes any U/Th depth sampling error. The ChronMean is nearly identical to our parabolic fit for stalagmite GU-Xi-1 from 1750 onwards giving us confidence in our age chronology and timing of the isotopes events to the volcano chronology. Furthermore, there is supporting evidence that some stalagmites grow in a parabolic fashion. Parabolic growth of speleothems has been previously noted [52] and may be a natural function of conical growth. Finally, the similarity of our record with that from another stalagmite from MesoAmerica [17] ( Fig. 6 ) increases our confidence on the robustness of our age model. Samples and δ 18 O isotopic analysis 582 samples were continuously milled along the stalagmite growth axis of GU-Xi-1 stalagmite using a digitally controlled micro-milling machine (SHERLINE 5410). Samples were milled at 0.3 mm intervals ( Fig. 2a ) giving a temporal resolution ranging between yearly at the top and seasonal at the bottom. Growth rate of the speleothem fluctuated from ∼ 1–3 mm per year. The samples were analyzed using a continuous flow isotope ratio mass spectrometry [53] at the ETH Zurich, Switzerland. Details on the methodology are given in ref. 53 . MS2 was used as in-house reference material (powdered Carrara marble, MS2 [53] ), with isotope ratios ( 18 O/ 16 O and 13 C/ 12 C) reported in standard Delta notation relative to the Vienna Pee Dee Belemnite (% VPDB) standard (see Supplementary data 1 ). The external analytical precision for δ 18 O is better than 0.06%. Amount effect The amount effect on stalagmites has been rigorously studied for Mesoamerica and has shown to be valid [15] , [16] . The comparison between precipitation and δ 18 O in Fig. 3 indicates that the speleothem’s oxygen isotopic properties capture the low-frequency variations of rainfall outside the cave, with the proportion of heavy isotope inversely proportional to the amount of precipitation. Observational datasets The precipitation data are from the University of East Anglia—Climate Research Unit gridded historical Time Series version 3.21 for 1901–2012 (for more information, see: http://badc.nerc.ac.uk/view/badc.nerc.ac.uk__ATOM__ACTIVITY_0c08abfc-f2d5-11e2-a948-00163e251233 ). The SST data are from the NOAA National Climate Data Center Extended Reconstructed Sea Surface Temperature analysis [54] version 3b averaged over the summer months between 1901 and 2012 in Fig. 4a , and between1880 and 2006 in Fig. 4c to fit with the length of the observed precipitation and δ 18 O records, respectively. The SLP data are from the NOAA Environmental Research Laboratories Twentieth Century Reanalysis Project [55] version 2, covering the period between 1901 and 2006 in Fig. 4b and between 1880 and 2006 in Fig. 4d . The SLP data were averaged over the winter (December–March) preceding the summer, as this is when the atmosphere forces the SST pattern seen in Fig. 4a [10] . Support for the Twentieth Century Reanalysis Project dataset was provided by the US Department of Energy, Office of Science Innovative and Novel Computational Impact on Theory and Experiment program and Office of Biological and Environmental Research and by the National Oceanic and Atmospheric Administration Climate Program Office. Data for Belize-City precipitation is from the National Oceanic and Atmospheric Administration, monthly Global Historical Climatology Network ( http://www.ncdc.noaa.gov/ghcnm/ ). Simulated precipitation datasets Time series of Yucatán precipitation covering the period 1700–2005 were obtained from an ensemble of climate model simulations from the repository of the Coupled Model Intercomparison Project 5. For each model, the time series were created by merging the data from the last-millennium simulation (past1000, which ends in 1849) with the corresponding data from one of the historical simulations (starting in 1850). Yucatán is defined as the area between 91°W and 87°W and between 16°N and 22°N (all model data were interpolated to a 2° × 2° grid before selecting the region). Volcanic forcing estimates Forcing estimates from ECHAM5/MPIOM [56] and Bergen Climate Model [28] are derived from volcanic forcing-only and natural (volcanic and solar) last-millennium simulations, respectively. Forcing estimates for CCSM4 [57] are derived from the full-forcing last-millennium simulation available in the Coupled Model Intercomparison Project 5 repository. Long-term influences from greenhouse gases in CCSM4 are accounted for by removing the fourth-order polynomial trend over the period 1750–2005. Natural forcing was then estimated based on clear-sky top-of-atmosphere radiative fluxes to discard cloud related feedbacks. The simulations use different reconstructions of aerosol optical properties for volcanic forcing: ECHAM5/MPIOM uses the reconstruction by [58] ; Bergen Climate Model uses the reconstruction by [59] ; CCSM4 uses the reconstruction by [60] . Cumulative volcanic forcing is obtained by cumulatively adding the forcing of each volcanic event through time. Statistical significance Statistical significance for correlations accounts for the effective degrees of freedom based on autocorrelation following the method by [61] . The lag in Fig. 3 was determined based on a cross-correlation analysis between the two time series with lags varying between −10 and +10 years. The binomial smoothed 71-year precipitation record shown in Fig. 3 has 15 degrees of freedom, so that a correlation value of 0.43 is significant at the 95% level using a directional test (appropriate in this case as we can surmise that the precipitation is the driver of the δ 18 O variations and not vice versa). Wavelet analysis Wavelet coherence spectra were calculated using the tool by ref. 62 . For additional information, see ref. 63 . The power of the wavelet coherence spectrum can be interpreted as a measure of the strength of the local (in the time-frequency domain) correlation between the two time series. How to cite this article : Winter, A. et al. Persistent drying in the tropics linked to natural forcing. Nat. Commun. 6:7627 doi: 10.1038/ncomms8627 (2015).